Ribosomal protein S1 functions as a termination factor in RNA synthesis by Qβ phage replicase S1 is the largest ribosomal protein, and is vitally important for the cell. S1 is also a subunit of Qβ replicase, the RNA-directed RNA polymerase of bacteriophage Qβ. In both protein and RNA syntheses, S1 is commonly believed to bind to a template RNA at the initiation step, and not to be involved in later events. Here, we show that in Qβ replicase-mediated RNA synthesis, S1 functions at the termination step by promoting release of the product strand in a single-stranded form. This function is fulfilled by the N-terminal fragment comprising the first two S1 domains. The results suggest that S1 might also have a role other than mRNA binding in the ribosome. Qβ replicase is an enzyme most efficiently amplifying RNA in vitro [1] . By reading a single-stranded RNA template, Qβ replicase synthesizes the complementary single-stranded RNA product [2] . In the next replication round, both of the strands serve as templates for the synthesis of their complementary copies, and so on. Thus, the number of templates doubles in each round, and increases exponentially as long as the replicase remains in molar excess over RNA [3] . Overall, the process resembles PCR [4] , except unlike PCR, it occurs under isothermal conditions, at physiological temperature, as there are no double-stranded products that need to be melted. Qβ replicase consists of four different subunits, one of which (β) is encoded by the phage genomic RNA [5] , [6] and the other three are host ( Escherichia coli ) proteins involved in protein synthesis: ribosomal protein S1 [7] , [8] , [9] and elongation factors EF-Tu and EF-Ts [10] . While the roles of the elongation factors remain unclear, the function of S1 in Qβ replicase seemed to be well established as long as 40 years ago, when it was for the first time separated from the three-subunit core enzyme [7] . Since then, it was commonly accepted that S1 (i) is required for copying the phage genomic (plus) strand RNA; (ii) triggers initiation of RNA synthesis by specifically binding to this template; (iii) is not involved in later events in the replication cycle; and (iv) is not needed for the copying of other Qβ replicase templates, including the Qβ RNA minus strand and non-genomic small replicable RNAs (‘6S’ or RQ RNAs, for ‘Replicable by Qβ replicase’) [7] , [11] , [12] , [13] , [14] . Ascribing to S1 a role at the initiation step is congenial with the traditional view of S1 as an RNA-binding protein whose function is attracting single-stranded RNA [15] . In the E. coli ribosome, S1 is thought to be involved in the initiation of protein synthesis by capturing mRNA [15] and/or unwinding the mRNA secondary structure [16] , [17] . The S1 sequence contains six OB ( O ligonucleotide/oligosaccharide B inding) motifs presumably corresponding to distinct structural domains [18] , [19] ; of these, the first two were implicated in binding with the ribosome [20] and Qβ replicase [21] , whereas the middle two possess affinity to RNA [15] . Here, we show that none of the above statements regarding the role of S1 in Qβ replicase is correct. In particular, we demonstrate that S1 is dispensable for one-round copying of any template, but ensures exponential amplification of either Qβ RNA or RQ RNA by promoting release of the product strand in a single-stranded form. In this function, S1 can be replaced by its fragment comprising the first two OB motifs. The results suggest that in the ribosome too, S1 might have a role other than binding of mRNA during initiation of its translation. S1 is needed for efficient replication of RQ RNA In the course of studies on functional properties of the core enzyme, we discovered that, in contrast to the common belief, the rate and yield of the exponential amplification of an RQ RNA, a 140-nucleotide (nt)-long variant of non-genomic RQ135 RNA [22] , dramatically increased upon the addition of equimolar amount of protein S1 ( Fig. 1a ). In agreement with the earlier report [7] , the stimulatory action of S1 was weak, if any, when the same RNA was amplified linearly, that is, when the RNA concentration equalled or exceeded that of replicase, and at copying poly(C) ( Supplementary Fig. S1 ). 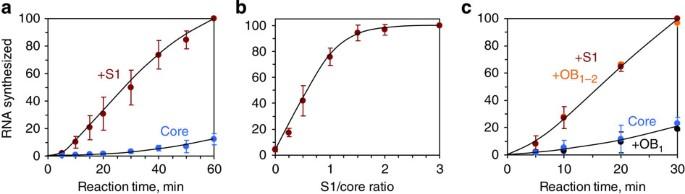Figure 1: Effect of protein S1 and its fragments on the replication of RQ RNA. Initially, reactions contained 1.66 nM RQ135 RNA and 360 nM Qβ replicase core. Plotted are amounts of full-sized product strands expressed as per cent of the maximum value attained in a particular experiment in the presence of S1. Shown are mean values; error bars represent ranges of data fromnindependent experiments. (a) Time course of RNA synthesis in the absence or presence of 360 nM S1;n=4. (b) RNA synthesized by the 10th min at varied S1-to-Qβ replicase core ratio;n=3. (c) Time course of RNA synthesis by the core enzyme alone or combined with 360 nM S1 or its fragment OB1or OB1–2;n=2. Figure 1: Effect of protein S1 and its fragments on the replication of RQ RNA. Initially, reactions contained 1.66 nM RQ135 RNA and 360 nM Qβ replicase core. Plotted are amounts of full-sized product strands expressed as per cent of the maximum value attained in a particular experiment in the presence of S1. Shown are mean values; error bars represent ranges of data from n independent experiments. ( a ) Time course of RNA synthesis in the absence or presence of 360 nM S1; n =4. ( b ) RNA synthesized by the 10th min at varied S1-to-Qβ replicase core ratio; n =3. ( c ) Time course of RNA synthesis by the core enzyme alone or combined with 360 nM S1 or its fragment OB 1 or OB 1–2 ; n =2. Full size image The observed stimulation by S1 of the exponential replication of RQ RNA could be attributed to either stabilization of vacant Qβ replicase molecules, which were in excess initially, and therefore to a higher specific activity of the enzyme late in the reaction, and/or to enhanced initiation due to increased affinity of Qβ replicase for the RNA template because of the RNA-binding capacity of S1, the result being accumulated in a number of successive rounds. The first possibility was eliminated by the experiment in Supplementary Fig. S2a showing that S1 did not influence inactivation of Qβ replicase in the absence of ligands. To explore the second possibility, we used the earlier reported protocol [23] to measure time course of initiation in the presence and absence of S1, taking advantage of the ability of aurintricarboxylic acid to stop initiation without affecting elongation of the initiated strands [24] . Initiation, including the synthesis of a short oligo(G) primer, occurred during incubation of the enzyme with RNA template and GTP. At specified time points, aurintricarboxylic acid was added along with the missing NTPs. After the initiated strands were allowed to be elongated to the length of the template, the products were separated by gel electrophoresis and the amount of the full-sized product strands was determined. Although S1 slightly increased the rate and yield of initiation on RQ RNA (reflected by the slope and plateau of the curves, respectively; Fig. 2a , left panel), the effect was too weak to account for the observed enhancement of the exponential replication ( Fig. 1a ). Moreover, S1 did not affect stability of the initiation complex ( Supplementary Fig. S2b ). 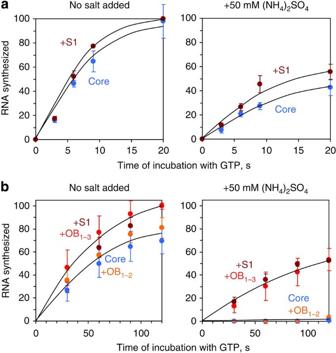Figure 2: Effect of protein S1 and its fragments on the initiation of RNA synthesis. After incubation for the indicated time intervals with 1 mM GTP, in the presence or absence of 50 mM ammonium sulfate, of (a) 0.1 μM RQ135 RNA or (b) 0.1 μM Qβ RNA with 1 μM replicase core alone or combined with 1 μM of S1 or its fragment OB1–2or OB1–3, the other three NTPs and aurintricarboxylic acid were added to the final concentrations of 0.1 and 1 mM, respectively, and reactions were incubated for additional 10 min to elongate the initiated strands. Plotted are amounts of full-sized product strands expressed as per cent of the maximum value attained in a particular experiment in the presence of S1 without the addition of ammonium sulfate. Shown are mean values; error bars represent ranges of data from three independent experiments. Figure 2: Effect of protein S1 and its fragments on the initiation of RNA synthesis. After incubation for the indicated time intervals with 1 mM GTP, in the presence or absence of 50 mM ammonium sulfate, of ( a ) 0.1 μM RQ135 RNA or ( b ) 0.1 μM Qβ RNA with 1 μM replicase core alone or combined with 1 μM of S1 or its fragment OB 1–2 or OB 1–3 , the other three NTPs and aurintricarboxylic acid were added to the final concentrations of 0.1 and 1 mM, respectively, and reactions were incubated for additional 10 min to elongate the initiated strands. Plotted are amounts of full-sized product strands expressed as per cent of the maximum value attained in a particular experiment in the presence of S1 without the addition of ammonium sulfate. Shown are mean values; error bars represent ranges of data from three independent experiments. Full size image Initiation requires S1 only in high-salt buffer The concept that S1 is exclusively needed for initiation on the Qβ(+) RNA and is not needed for initiation on other templates was based on data obtained in a high-salt buffer [7] . The authors argued that salt helped to avoid the interfering ‘spontaneous’ RNA synthesis that was later shown to be caused by traces of contaminating RQ RNAs [25] . Further, the authors of the concept measured the total RNA synthesis rather than the initiation resulting in the full-sized template-specific products; they assumed that S1 promoted the synthesis through enhanced initiation, but neither they nor others ever tested this hypothesis directly. It was therefore important to check whether S1 affects initiation on the Qβ(+) RNA, whether this effect is different from the one seen with RQ RNA, and whether high salt modulates the S1 action. Contrary to the expectation, initiation on the Qβ(+) RNA in the standard low-salt buffer depended on S1 almost as weakly as did initiation on RQ RNA (cf. Fig. 2a , left panels). Addition of 50 mM ammonium sulfate in the presence of S1 inhibited initiation on each of the templates to roughly the same extent, approximately two-fold ( Fig. 2a , brown symbols). However, the absence of S1 resulted in a nearly total suppression by the salt of initiation on the Qβ(+) RNA, whereas marginally affected initiation on RQ RNA (cf. brown and blue symbols on Fig. 2a , right panels). Thus, S1 indeed stimulates initiation on the Qβ(+) RNA and not on RQ RNA, but this stimulation is observed in the special case of a high-salt buffer only. S1 reduces the proportion of double-stranded RNA Although not seen at monitoring the total RQ RNA synthesis in the linear mode ( Supplementary Fig. S1a ), the effect of S1 became apparent when the reaction products were analyzed by gel electrophoresis, which revealed a greater proportion of single-stranded RNA in the presence of S1 ( Fig. 3a ). This could help explaining the much higher replication rate in the exponential mode ( Fig. 1a ), as only single-stranded RNA would be utilized by Qβ replicase as a template in the subsequent rounds of synthesis [2] . 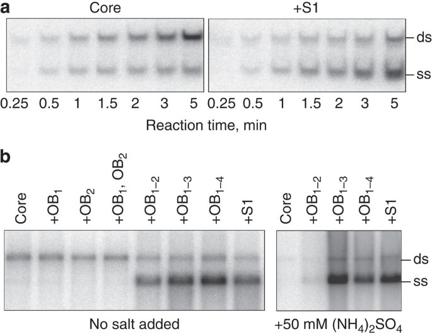Figure 3: Effect of S1 and its fragments on the accumulation of single-stranded products. The single-stranded (ss) and double-stranded (ds) phenol-extracted32P-labeled reaction products were separated by gel electrophoresis. (a) Time course of replication of RQ135 RNA (140 nt) in the absence or presence of S1. Initially, reactions contained 0.1 μM each of RQ135 RNA, core replicase, and S1 (where indicated). (b) Products synthesized during 30 min on Qβ(+) RNA (4217, nt) by the replicase core alone or in combination with S1 or its fragments in the absence or presence of 50 mM ammonium sulphate. Figure 3: Effect of S1 and its fragments on the accumulation of single-stranded products. The single-stranded (ss) and double-stranded (ds) phenol-extracted 32 P-labeled reaction products were separated by gel electrophoresis. ( a ) Time course of replication of RQ135 RNA (140 nt) in the absence or presence of S1. Initially, reactions contained 0.1 μM each of RQ135 RNA, core replicase, and S1 (where indicated). ( b ) Products synthesized during 30 min on Qβ(+) RNA (4217, nt) by the replicase core alone or in combination with S1 or its fragments in the absence or presence of 50 mM ammonium sulphate. Full size image Qualitatively similar electrophoresis pattern was obtained with the Qβ(+) RNA too. In the absence of S1, a labeled product was formed that co-migrated with the double-stranded Qβ RNA, suggesting that a full-sized minus strand was synthesized that annealed with the unlabeled template. In contradistinction, there was also a large amount of single-stranded product in the presence of S1 ( Fig. 3b ). Thus, contrary to the common belief, S1 turned out to be dispensable for a one-round copying of the Qβ(+) RNA. However, mostly, a double-stranded product was formed in the absence of S1. It looked as if S1 either helped the product strand to stay single-stranded or unwound its duplex with the complementary template. Each of these possibilities seemed plausible in view of S1’s ability of binding to a single-stranded RNA and unwinding a double-stranded RNA [15] , [16] , [17] . The patterns of Fig. 3 might have been distorted by the phenol extraction of samples before electrophoresis, which could cause conversion of single-stranded replicative complexes into the double-stranded form [26] . The true proportion of single-stranded and double-stranded forms can be determined by digesting the reaction products with a single-strand-specific ribonuclease prior to phenol extraction [27] . The results of such an assay showed that indeed, the core replicase produced mainly double-stranded RNA, whereas the holoenzyme produced mostly single-stranded product ( Fig. 4a ). 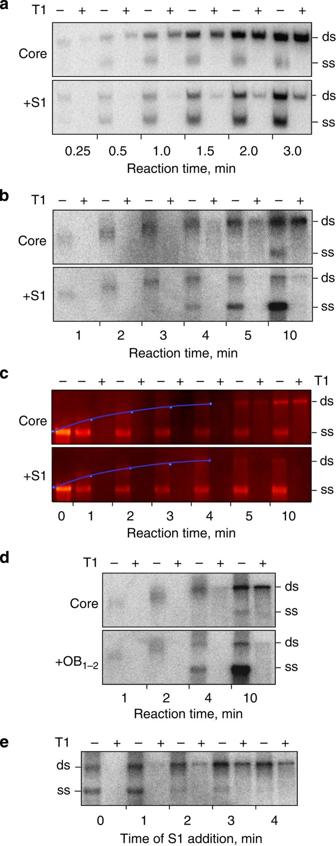Figure 4: Effect of S1 and OB1-2on product strand release and strandedness of the replicative complex. 32P-labeled replication products were either digested (lanes ‘+’) or not (lanes ‘−’) with ribonuclease T1 (capable of cleaving single-stranded, and not double-stranded RNAs47) prior to phenol extraction and gel electrophoresis. (a) Time course of replication of RQ135 RNA (140 nt) in the absence or presence of S1 carried out as inFig. 3a. At the indicated time points, the reactions were stopped by the addition of 10 μl of 20 mM EDTA containing or not 100 U of ribonuclease T1, and further incubated at 22 °C for 2 min. (b) Time course of replication of Qβ(+) RNA (4217, nt) by the replicase core alone or in combination with S1. Here and below, samples in lanes ‘+’ were mixed at the indicated time points with 1 μl of 100 U μl−1ribonuclease T1 and further incubated for 15 s at 30 °C. (c) The same gel as in (b) stained with ethidium bromide. Blue dots indicate median position of bands comprising the nascent product strands annealed with the template. (d) Time course of Qβ(+) RNA replication by the replicase core alone or in combination with fragment OB1–2. (e) Products of a 5-min Qβ(+) RNA replication by the replicase core enzyme to which S1 was added at the indicated time points. Figure 4: Effect of S1 and OB 1-2 on product strand release and strandedness of the replicative complex. 32 P-labeled replication products were either digested (lanes ‘+’) or not (lanes ‘−’) with ribonuclease T1 (capable of cleaving single-stranded, and not double-stranded RNAs [47] ) prior to phenol extraction and gel electrophoresis. ( a ) Time course of replication of RQ135 RNA (140 nt) in the absence or presence of S1 carried out as in Fig. 3a . At the indicated time points, the reactions were stopped by the addition of 10 μl of 20 mM EDTA containing or not 100 U of ribonuclease T1, and further incubated at 22 °C for 2 min. ( b ) Time course of replication of Qβ(+) RNA (4217, nt) by the replicase core alone or in combination with S1. Here and below, samples in lanes ‘+’ were mixed at the indicated time points with 1 μl of 100 U μl −1 ribonuclease T1 and further incubated for 15 s at 30 °C. ( c ) The same gel as in ( b ) stained with ethidium bromide. Blue dots indicate median position of bands comprising the nascent product strands annealed with the template. ( d ) Time course of Qβ(+) RNA replication by the replicase core alone or in combination with fragment OB 1–2 . ( e ) Products of a 5-min Qβ(+) RNA replication by the replicase core enzyme to which S1 was added at the indicated time points. Full size image S1 can be replaced by its first two domains To check whether the RNA-binding or helix-unwinding ability of S1 contributed to the observed effects, we prepared a series of nested N-terminal S1 fragments containing 1–4 of the total six OB motifs ( Supplementary Fig. S3 ) and tested them for the ability to functionally replace S1, bearing in mind that the third and the forth motifs harbor the RNA-binding site [28] and are therefore required for the unwinding activity [15] . To our surprise, fragment OB 1–2 only containing two first OB motifs stimulated replication of both RQ RNA ( Fig. 1c ) and Qβ RNA ( Fig. 3b , left panel) in the standard low-salt reaction buffer as efficiently as did the full-sized S1, although it did not form detectable complexes with RNA ( Supplementary Fig. S4 ). Earlier, this fragment was shown to be responsible for the binding of S1 with Qβ replicase [21] . In contrast, fragment OB 1–2 failed to substitute for S1 in a high-salt buffer, whether in initiation ( Fig. 2b ) or in replication ( Fig. 3b , right panel). In its anti-salt action, S1 could entirely be replaced by fragment OB 1–3 containing the first three OB motifs ( Figs 2b and 3b , right panel). Unlike fragment OB 1–2 , fragment OB 1–3 showed affinity for RNA in a gel-shift test, albeit an order of magnitude weaker than did the full-sized S1 ( Supplementary Fig. S4 ). It should be noted that, in addition to OB 1–2 , fragment OB 1–3 contains the third OB motif, one of the two RNA-binding domains [15] , which seems to confer on the fragment the affinity for RNA. S1 is not needed during elongation of the nascent strand The length of the Qβ(+) RNA (4217, nt (ref. 14 ), ≈30 times larger than that of RQ135 RNA) allowed us to monitor the growth of the complementary minus strand. Figure 4b shows the result of such an experiment. The 32 P-labeled products synthesized by specified time points were either treated or not with ribonuclease, extracted with phenol, and then separated by electrophoresis through agarose. In the untreated samples, the nascent product strand became annealed with the unlabeled template upon phenol extraction, and hence, migrated between the single-stranded and double-stranded Qβ RNA: the longer the nascent strand, the lower its mobility. Therefore, untreated samples (lanes ‘−’) enabled monitoring the strand elongation; this can most conveniently be done on an ethidium bromide-stained image ( Fig. 4c ). To facilitate location of the nascent strand/template hybrids at different time points, the respective bands in Fig. 4c were marked with blue dots. It is seen that whether or not was S1 present during elongation, the dots fit into the same curve indicating that S1 does not appreciably influence the rate of elongation. Samples treated with ribonuclease (lanes ‘+’) enabled assessment of the single-strandedness of the nascent strand (and hence of the replicative complex): only double-stranded RNA would survive the treatment. It is seen that product RNA remained sensitive to ribonuclease both in the presence and absence of S1 during the entire elongation phase ( Fig. 4b ). It follows that S1 is needed neither for the elongation of nascent strands, nor for maintenance of the elongating replicative complex single-stranded. S1 promotes release of the product strand In the presence of S1, the labeled single-stranded product RNA began to release from the replicative complex (and therefore became nonannealeable with the template at phenol extraction) soon after completion of the elongation, by the 4th min ( Fig. 4b ‘+S1’, lanes ‘–’), whereas in the absence of S1, a similar amount of the single-stranded product was only released by the 10th min ( Fig. 4b ‘core’, lanes ‘–’), with most of the replicative complex having been collapsed by this time into a ribonuclease-insensitive duplex ( Fig. 4b ‘core’, lanes ‘+’). It follows that S1 increases the rate of the product-strand release after elongation [29] , that is, functions as RNA release factor at the termination step, thereby accelerating the replicase turnover and preventing spontaneous annealing of the complementary template and product strands that are kept close to each other in the unterminated replicative complex. The fragment OB 1–2 acts similarly ( Fig. 4d ). S1 added before completion of elongation rescues replication The conclusion that S1 functions at the termination step was further substantiated by the observation that it performed its product strand release function even if added to the core enzyme after initiation and before the completion of elongation at about 3 min from the reaction onset ( Fig. 4e ). If S1 was added later, it could not catalyze the product strand release, and the replicative complex collapsed into duplex upon further incubation even if it remained single-stranded at the time of S1 addition. For example, in the reaction performed by the core enzyme, the product remained entirely sensitive to ribonuclease by the 3rd min ( Fig. 4b ‘core’, lanes ‘+’). However, if the reaction received S1 at this time point and further incubated for the total of 5 min, the sensitivity of the product to ribonuclease decreased to roughly the same degree as it did by the 5th min when S1 was not added at all (cf. the 3-min point of Fig. 4e and 5-min point of Fig. 4b ‘core’). S1 promotes termination during Qβ RNA minus strand copying It is commonly adopted that, at replication of the Qβ phage RNA, S1 is only needed for copying the plus strand, and not the minus strand [7] , [11] , [12] , [13] , [14] . To check this issue, we explored effects of S1 on copying the transcript synthesized from a plasmid carrying the Qβ(−) cDNA under the T7 promoter [30] . 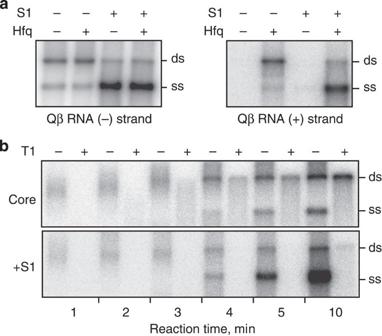Figure 5: Effect of protein S1 on copying the Qβ RNA minus strand. (a) Products synthesized during 30 min on the Qβ(−) and (+) RNAs (4,217 nt each) in the presence or absence of S1 and Hfq (host factor). (b) Time course of the Qβ(−) RNA replication in the absence of Hfq by the replicase core alone or in combination with S1. Experimental conditions were as inFig. 4b. Figure 5a demonstrates that the transcript is indeed the minus strand as, in contrast to the plus strand, it is copied by Qβ replicase independently of the host factor (protein Hfq) [31] ; yet the effects of S1 on copying the two templates is the same: in each case, S1 promotes accumulation of the single-stranded RNA and reduces the proportion of double-stranded RNA in the reaction products. Figure 5b further shows that, as with the plus strand, S1 does not affect the elongation phase and single-strandedness of the replicative intermediate during copying the minus strand, but promotes release of the synthesized plus strand after elongation. Figure 5: Effect of protein S1 on copying the Qβ RNA minus strand. ( a ) Products synthesized during 30 min on the Qβ(−) and (+) RNAs (4,217 nt each) in the presence or absence of S1 and Hfq (host factor). ( b ) Time course of the Qβ(−) RNA replication in the absence of Hfq by the replicase core alone or in combination with S1. Experimental conditions were as in Fig. 4b . Full size image In their pioneering work, Weissmann et al . [7] had reported that, when assayed in a buffer to which 100 mM CsCl or KCl was added in order to suppress the interfering synthesis of RQ RNAs, the RNA synthesis on the Qβ(+) RNA was absolutely dependent on the presence of the Qβ replicase α subunit, later identified as the ribosomal protein S1 [8] , [9] . When the salt was not added, some synthesis occurred in the absence of α subunit, yet it was stimulated 10-fold upon the addition of S1. Almost no dependence on S1 was observed with other templates tested, including poly(C), RQ RNAs and Qβ(−) RNA. The authors concluded that unlike other templates, Qβ(+) RNA has a low intrinsic affinity for α-less Qβ replicase (the core enzyme), which is further reduced at high ionic strength, and that S1 is needed for tight binding of this template by the enzyme. Later, this statement has acquired a stronger form; namely, that S1 is only required for binding Qβ(+) RNA to the replicase at the initiation step, and that even with this RNA, elongation and termination steps are not altered by S1 [12] . Other authors also concluded that S1 solely functions at initiation of the Qβ(+) RNA copying [32] , [33] . Our data confirm some observations of Weissmann et al . [7] ; in particular, the dependence on S1 of copying the Qβ(+) RNA strand in a high-salt buffer and independence on S1 of copying poly(C) and replication of RQ RNA (in the linear mode). However, in our experiments, both initiation and single-round copying of the Qβ(+) RNA were largely independent of S1 in a low-salt buffer, whereas replication of RQ RNA proved to be strongly dependent on S1 if assayed in the exponential mode. Separate monitoring of single-stranded and double-stranded RNAs in the reaction products revealed the reason for such paradoxical results. S1 essentially prevents the formation of double-stranded RNAs, thereby conferring on Qβ replicase a feature critically important for its ability [2] , [26] of exponentially amplifying RNA in the absence of double-stranded intermediates. Surprisingly, this function of S1 does not utilize its known abilities of binding single-stranded RNAs [15] , [34] and unwinding RNA duplexes [16] , [17] . Moreover, Qβ replicase core itself is able to maintain the single-strandedness of the replicative intermediate during the entire elongation phase. After completion of elongation, in the absence of S1, the full-sized product strand begins to slowly anneal to the template, with only a small fraction being spontaneously released single-stranded; whereas in the presence of S1, the product strand rapidly dissociates from the replicative complex. It follows that S1 promotes termination of RNA synthesis, and this seems to be the main function of S1, equally important for any template capable of exponential amplification by Qβ replicase. Moreover, S1 can perform its terminating function even if added during elongation, but not after that. Our data show that there is a ‘no-return point’ somewhere at the end of elongation after which the replicative complex cannot be rescued by extraneous S1. What could that point be? During initiation on a legitimate template, Qβ replicase undergoes GTP-triggered transition into a closed conformation, from which neither the template nor the product strand can dissociate until the full-sized product is synthesized [35] . Being advantageous for elongation of the initiated strands, the closed conformation must become an obstacle for the continuation of replication after elongation. To enable product strand release, a reverse transition to the initial (open) conformation must occur at the termination step. We hypothesize that the reverse transition is triggered by the non-templated adenylylation of the 3′-terminal oligo(C) known to occur at termination of every legitimate product strand [12] , [36] , and that S1 needs to build into the replicative complex before this transition to be able of catalyzing the product strand release. Further experiments are needed to check this hypothesis. The finding that protein S1 functions as termination factor does not undermine its role during initiation. Besides stimulating initiation on the Qβ(+) RNA in a high-salt buffer, S1 might promote re-initiation, at least by providing both the original template and the newly synthesized product strand in the single-stranded form. No doubt, S1 has an important role in vivo during de novo initiation on the phage RNA strand that has infected the cell, when it helps the newly synthesized replicase to free the strand of the translating ribosomes [37] by binding upstream of the coat protein cistron [38] . S1 is the largest ribosomal protein that has also been implicated in a number of cellular functions other than protein synthesis [39] . Amber mutation [40] or deletion [41] of S1 is lethal, suggesting that S1 is vitally important to the cell. In this report, we demonstrate that the main function of S1 in the RNA synthesis by Qβ replicase is displacing RNA away from the replicase complex. This finding changes the S1 paradigm and provokes re-examination of the role of this protein in other instances, including its functioning in the ribosome. For many years, the role of S1 in translation was considered to be mRNA binding to the ribosome at the initiating step. However, this concept did not explain why, unlike initiation factors, S1 is present in the ribosome in stoichiometric amounts and stays bound to the ribosome after completion of the initiation step [15] . Assuming that Qβ replicase employs the function that has already evolved for the use in protein synthesis, one might speculate that, apart from enhancing the mRNA binding, S1 might also promote release of single-stranded RNAs (mRNA and/or tRNAs) from the ribosome. Finally, this paper shows that in Qβ replicase, the RNA release during termination and anti-salt function during initiation are entirely fulfilled by S1 fragments comprising the first two and three OB motifs, respectively. The assignment of clear-cut functions to particular S1 domains will advance future structural and functional studies of both Qβ replicase and the ribosome. Templates The used variant of RQ135 RNA was prepared by transcription of Sma I-digested plasmid pT7RQ135 –1 (–) [42] modified by inserting CGAUCC between positions 52 and 53 of the original RQ135 –1 (–) sequence; the template properties of this variant were indistinguishable [35] from those of the authentic RQ135 RNA [22] . Qβ(+) RNA was isolated from purified wild-type phage particles lysed with SDS, followed by centrifugation through a 15% sucrose cushion and phenol extraction [25] . Qβ(−) RNA was prepared by transcription of SmaI-digested plasmid pQβ8 [30] . Reaction conditions and product analysis Unless otherwise indicated, all reactions were run in 10 μl of the reaction buffer (100 mM HEPES-NaOH pH 7.5, 10 mM MgCl 2 , 1 mM EDTA, 0.1% Triton X-100) at 30 °C, in the presence of 1 mM each of NTPs. The reactions were stopped by the addition of 10 μl of 20 mM EDTA, treated or not with ribonuclease T1 as indicated, extracted with 20 μl of phenol/chloroform (1:1, v/v), and 10 μl of the aqueous phase was subjected to non-denaturing electrophoresis through a 8% polyacrylamide gel [35] in case of RQ RNA or 1% agarose gel in case of Qβ RNA. The 32 P-labeled RNA bands on dried gels were revealed using a Cyclone phosphor storage system (Packard Instrument) and either presented here as original images, or quantified by measuring the band intensities [43] . In experiments with the Qβ(+) RNA, the reaction mixture contained 0.1 μM RNA template, 1 μM core replicase, 0.1 μM E. coli Hfq (host factor for phage Qβ) and, where indicated, 1 μM protein S1 or its fragment. Synthesis on Qβ(−) RNA was studied similarly, but except otherwise indicated, Hfq was not added. S1-free Q replicase core E. coli BL21 (DE3) cells co-transformed with plasmids pET-TsE-TuE encoding E. coli elongation factors EF-Tu and EF-Ts under the control of T7 promoter and pBAD-REP encoding the β subunit under the control of the E. coli ara BAD arabinose operon promoter (P BAD ) and protein AraC ( Supplementary Methods ) were grown in the LB medium containing 100 μg ml −1 ampicillin, 50 μg ml −1 kanamycin and 1 mM D (+)-lactose at 30 °C in 5-l flasks with shaking at 150 r.p.m. until the optical density of ≈2 at 600 nm. Synthesis of the replicase β-subunit was then induced by adding L (+)-arabinose to 0.2% (w/v), and the growth was continued for another 3 h. Cells were harvested by centrifugation for 20 min at 4,000 r.p.m. in a centrifuge J-6B Swinging Bucket Rotor (Beckman) at 4 °C, then frozen and stored at −20 °C until use. The yield was about 5 g of cell paste per 1 l of culture; co-expression of the two plasmids provided for accumulation in the cells of large amounts of soluble Qβ replicase without precipitation of the β subunit. For the enzyme isolation, 10 g of the cell paste was thawed, suspended in 20 ml of the lysis buffer (50 mM Tris-HCl pH 7.5, 500 mM NaCl, 50 mM MgCl 2 , 1 mM EDTA, 7 mM 2-mercaptoethanol, 1 mM phenylmethylsulfonyl fluoride), and disrupted with an Ultrasonic Homogenizer 4710 (Cole-Parmer) in a beaker continuously cooled in an ice bath. Four rounds of sonication were performed with the power switch set to 7, each round being 30–40 s with 1.5–2 min intervals in between. To the lysate, 0.9 ml of a 10% polyethyleneimine-HCl (pH 7.5) was added dropwise with vigorous stirring, which then continued for another 20 min. The precipitate formed was removed along with the cell debris at 10,000 g in Centrifuge 2804r (Eppendorf) for 60 min at 4 °C. After a five-fold dilution with buffer TEM (50 mM Tris-HCl pH 7.5, 5 mM MgCl 2 , 1 mM EDTA, 7 mM 2-mercaptoethanol), the supernatant was applied to a 20-ml column of Q Sepharose High Performance (GE Healthcare Life Science) equilibrated with buffer TEM containing 0.1 M NaCl, and the protein was eluted with 250 ml of a linear gradient of 0.1–0.4 M NaCl in buffer TEM. To the combined fractions containing the replicase β-subunit (as determined by gel electrophoresis in SDS), a 4 M ammonium sulfate was added to a final concentration of 0.6 M. The sample was then applied to a 20-ml column of Butyl Sepharose High Performance (GE Healthcare Life Science) equilibrated in buffer TEM containing 0.8 M ammonium sulfate. The protein was eluted with 200 ml of a linear gradient of 0.8–0 M ammonium sulfate in buffer TEM. This completely separated the core enzyme from protein S1. To the combined fractions containing the replicase β-subunit and no protein S1, 5 M NaCl was added to a final concentration of 0.5 M. After reducing the volume to 1 ml in concentrator Vivaspin 20 MWCO 30,000 (GE Healthcare Life Science), the sample was subjected to gel filtration through a column of Superdex 200 HR 10/30 (GE Healthcare Life Science) equilibrated in buffer 20 mM Tris-HCl pH 7.5, 500 mM NaCl, 5 mM MgCl 2 , 1 mM EDTA and 7 mM 2-mercaptoethanol. Fractions whose absorption at 280 nm exceeded 50% of the peak value were pooled and concentrated to 30–35 mg/ml in Vivaspin 20 MWCO 30,000. The protein concentration was determined by measuring the sample absorbance at 280 nm using the value of A0.1%=0.767 calculated from the aminoacid composition of the core enzyme using the ProtParam tool ( au.expasy.org/tools/protparam.html ). The enzyme preparation was frozen in aliquots in liquid nitrogen and stored at −70 °C until use. Ribosomal protein S1 and its fragments Each of these proteins was isolated from E. coli cells transformed with a plasmid encoding S1 or its fragment ( Supplementary Methods ) that bore at the N terminus a His 6 tag followed by the recognition site for tobacco etch virus (TEV) protease [44] . E. coli BL21 (DE3) cells transformed with appropriate plasmid were grown with shaking at 150 r.p.m. during 16 h at 37 °C in the LB medium containing 100 mg l −1 ampicillin, 25 mM Na 2 HPO 4 , 25 mM KH 2 PO 4 , 10 mM (NH 4 ) 2 SO 4 , 2 mM MgSO 4 , 0.5% glycerol, 0.05% D (+)-glucose and 0.2% L (+)-lactose, and harvested as above. The yield was about 10 g of a cell paste per 1 l of culture. Overproduced S1 and its fragments accumulated in the cells in a non-soluble form; therefore, they were isolated in denatured state in urea and renatured as follows. Ten grams of a cell paste were suspended in 20 ml of the lysis buffer (20 mM Tris-HCl pH 8.0, 9.6 M urea, 7 mM 2-mercaptoethanol) and homogenized as above. Cleared lysate was loaded on a 5-ml Ni 2+ Sepharose HisTrap FF column (GE Healthcare Life Science), the column was washed with the lysis buffer containing 8 M urea, the adsorbed protein being renatured in situ by washing the column with a high-salt buffer (20 mM Tris-HCl pH 8.0, 0.5 M NaCl, 7 mM 2-mercaptoethanol), and then eluted with the same buffer supplemented with 250 mM imidazole. Fractions were analyzed by SDS electrophoresis through a 10% polyacrylamide gel, and those containing the desired protein were digested overnight at 4 °C with TEV protease, 1 mg of the protease being added per 50 mg of protein. This removed the His 6 tag and produced a protein whose N-terminal aminoacid was Gly ( Supplementary Fig. S3b ). After a 10-fold dilution of the digest with buffer TE (20 mM Tris-HCl pH 8.0, 1 mM EDTA, 7 mM 2-mercaptoethanol), a substantially pure protein were isolated by ion-exchange chromatography through a 20-ml column of Q Sepharose HP (GE Healthcare Life Science) using a linear gradient of 50–500 mM NaCl in buffer TE. If SDS electrophoresis showed notable impurities, the preparation was additionally purified by gel filtration through the Superdex 200 HR 10/30 column (see above) equilibrated in buffer 20 mM Tris-HCl pH 7.5, 150 mM NaCl, 5 mM MgCl 2 , 1 mM EDTA, 7 mM 2-mercaptoethanol. Protein concentration in the preparations obtained was determined by measuring their absorbance at 280 nm, using the values of A 0.1% calculated by ProtParam (see above): 0.777 (S1), 0.505 (OB 1 ), 0.372 (OB 1–2 ), 0.487 (OB 1–3 ), 0.727 (OB 1–4 ). As fragment OB 2 did not absorb at 280 nm, its amount was estimated by measuring the absorbance of a sample before digesting it with TEV protease, using the A 0.1% value of 0.162. The purified preparations were frozen in aliquots in liquid nitrogen and stored at −70 °C until use. Host factor Hfq was isolated from a 1 M NH 4 Cl ribosomal wash [45] by chromatography on poly(A) Sepharose [46] and freed of RNA by passing through a DEAE cellulose column in a buffer containing 8 M urea and 50 mM NaCl. How to cite this article: Vasilyev, N. N. et al . Ribosomal protein S1 functions as a termination factor in RNA synthesis by Qβ phage replicase. Nat. Commun. 4:1781 doi: 10.1038/ncomms2807 (2013).